Neural stem and progenitor cells shorten S-phase on commitment to neuron production During mammalian cerebral cortex development, the G1-phase of the cell cycle is known to lengthen, but it has been unclear which neural stem and progenitor cells are affected. In this paper, we develop a novel approach to determine cell-cycle parameters in specific classes of neural stem and progenitor cells, identified by molecular markers rather than location. We found that G1 lengthening was associated with the transition from stem cell-like apical progenitors to fate-restricted basal (intermediate) progenitors. Unexpectedly, expanding apical and basal progenitors exhibit a substantially longer S-phase than apical and basal progenitors committed to neuron production. Comparative genome-wide gene expression analysis of expanding versus committed progenitor cells revealed changes in key factors of cell-cycle regulation, DNA replication and repair and chromatin remodelling. Our findings suggest that expanding neural stem and progenitor cells invest more time during S-phase into quality control of replicated DNA than those committed to neuron production. During development of the mammalian cerebral cortex, neurons are generated from two principal classes of neural progenitor cells (NPCs). One class consists of somatic stem cell-like neuroepithelial cells and radial glial cells, collectively referred to as apical progenitors (APs), which exhibit apical–basal polarity, undergo mitosis at the ventricular (apical) surface, and the cell bodies of which constitute the ventricular zone (VZ) [1] , [2] , [3] , [4] . The second class consists of NPCs that originate from apical mitoses, translocate their cell bodies through the VZ in the basal direction, delaminate from the ventricular surface to form the subventricular zone (SVZ), downregulate apical–basal polarity (at least in rodents) and undergo mitosis in the basal VZ or SVZ [5] , [6] , [7] , [8] , [9] ; these NPCs are called basal progenitors (BPs) [2] or intermediate progenitor cells [4] . Regarding the balance between NPCs and neurons, there are three principal types of AP and BP divisions: self-expanding symmetric proliferative, self-renewing asymmetric BP- or neuron-generating, and self-consuming neurogenic [3] , [10] . The spatial organization of APs and BPs in M-phase is one key determinant of the type of NPC division [2] , [3] , [11] . Another key determinant is of a temporal nature. Specifically, concomitant with progression of neurogenesis, cell-cycle length of cortical NPCs in the VZ is known to increase [12] , [13] , [14] , and there are intriguing links between NPC cell-cycle length and neuron output [15] , [16] , [17] . NPC cell-cycle lengthening pertains specifically to the G1-phase [12] , [14] , [15] and can be a cause (rather than a consequence) of neurogenesis [16] , [17] , [18] . Conversely, reducing cell-cycle length, specifically G1, of NPCs in the cerebral cortex has recently been found to promote their expansion, with a transient delay in neurogenesis [19] , [20] . However, taking into account the coexistence of APs and newborn BPs in the VZ with the onset of neurogenesis, it is unclear whether cell-cycle lengthening of NPCs in the VZ, concomitant with the progression of neurogenesis, reflects the following: cell-cycle lengthening in an AP sub-population, as previously assumed [14] ; an increasing contribution, in the VZ, of newborn BPs, if these were to have a longer cell cycle than APs; or both. The second possibility is particularly relevant for consideration because, with progression of neurogenesis, an increasing proportion of APs switch to generate BPs [6] . In addition, determination of cell-cycle parameters of BPs is important per se . BPs, and SVZ progenitor cells in general, have been implicated in cortical expansion during evolution [21] , [22] . In rodents, BPs have been shown to undergo symmetric proliferative divisions, which result in their expansion, and symmetric neurogenic divisions, which result in their consumption [8] , [9] , [10] , [21] , [23] . It is thus of interest to determine whether proliferative and neurogenic BPs differ in their cell-cycle parameters. In the present study, we determined the cell-cycle parameters of BPs and compared them with APs, using cumulative labelling with thymidine analogues [24] . Compared with other approaches such as determining the time between two NPC divisions by live imaging in organotypic slice culture (for example, see ref. 20 ), cumulative labelling has the advantages of being carried out in vivo and providing information on individual cell-cycle phases. However, a prerequisite for this approach is a reliable means of identifying BPs. Determining the accumulation, in the SVZ, of interphase nuclei containing an S-phase label [25] , as was previously considered appropriate for APs by analysing interphase nuclei in the VZ [12] , may not be appropriate because, in the SVZ, BPs are intermingled with postmitotic neurons that inherit S-phase label from BPs, and a substantial proportion of BP nuclei in interphase, notably those of newborn BPs in G1, are located in the VZ, intermingled with AP interphase nuclei. Consequently, we have chosen to identify BP interphase nuclei and, for comparison, AP interphase nuclei, using molecular markers rather than SVZ versus VZ location. In the embryonic mouse cerebral cortex, virtually all apical mitoses, which by definition are APs [11] , [26] , are positive for Pax6, a transcription factor specifically expressed by neuroepithelial and radial glial cells and involved in their proliferation and neurogenesis [27] , [28] , [29] . Conversely, virtually all mitoses in the basal VZ and SVZ (collectively referred to as basal mitoses) are positive for the transcription factor Tbr2, a known marker of BPs [30] , [31] that controls the production of pyramidal neurons [32] , [33] . Given the availability of these molecular markers, in this study, we have developed a novel approach of determining cell-cycle parameters of APs and BPs by cumulative labelling with thymidine analogues. We find that BPs have a substantially longer G1-phase than APs, and that the previously observed G1 lengthening of neurogenic NPCs in the VZ [14] actually reflects the increasing contribution of BPs. Moreover, we used the antiproliferative gene Tis21 [34] , [35] , specifically Tis21 -GFP knock-in mouse embryos [6] , to distinguish neuronally committed from self-expanding APs and BPs, and find that the latter exhibit a substantially longer S-phase than the former, suggesting a greater time investment into quality control of replicated DNA in expanding NPCs. Identification of APs and BPs on the basis of molecular markers Our study investigates NPCs in the mouse E14.5 cerebral cortex. We first confirmed the previous observations [30] , [31] that Pax6 and Tbr2 [23] , [27] , [28] , [30] , [31] , [36] are expressed in virtually all apical and basal mitoses, respectively ( Supplementary Fig. S1 ). As described in Supplementary Note S1 , we identified AP or BP nuclei irrespective of their localization in the VZ or SVZ and defined Pax6-positive/Tbr2-negative (Pax6+/Tbr2−) interphase nuclei as AP nuclei, thereby excluding interphase nuclei of newborn BPs from the AP population. Similarly, we used the neuronal marker Tbr1 (ref. 30 ) to define Tbr2-positive/Tbr1-negative (Tbr2+/Tbr1−) interphase nuclei as BP nuclei, thereby excluding nuclei of neurons from the BP population. To determine the extent of intermingling of AP and BP interphase nuclei in the VZ and SVZ, and the proportion of APs committed to the neurogenic lineage, we performed triple immunofluorescence for Pax6, Tbr2 and Tis21 -GFP, which is specifically expressed in the sub-population of APs that generate neurons or neurogenic BPs [6] , [9] ( Fig. 1a ). With regard to APs, virtually all interphase nuclei in the VZ were Pax6+, as reported previously [27] , [30] , [31] . Counter immunofluorescence for Tbr2 revealed that ≈30% of Pax6+ interphase nuclei in the VZ were Tbr2+ ( Fig. 1b ), indicating that APs contributed ≈70% and newborn BPs ≈30% to VZ interphase nuclei ( Supplementary Fig. S2 ). 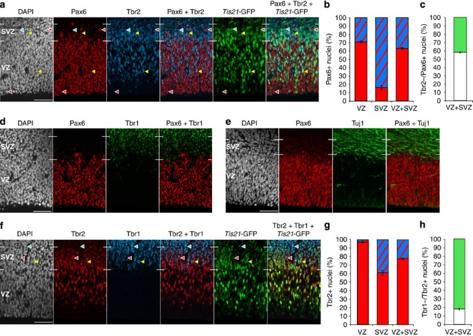Figure 1: Classification of proliferative and neurogenic APs and BPs on the basis of differential marker expression. (a) Pax6 (red), Tbr2 (blue),Tis21-GFP (green) and DAPI (white) staining. Red arrowheads, Pax6+/Tbr2−/Tis21-GFP− nuclei (APs); yellow arrowheads, Pax6+/Tbr2+/Tis21-GFP+ nuclei (BPs); blue arrowheads, Pax6−/Tbr2+/Tis21-GFP+ nucleus (BP). Scale bar, 50 μm. (b) Quantification of Tbr2+/Pax6+ (blue–red) and Tbr2−/Pax6+ (red) nuclei in VZ, SVZ and VZ+SVZ, each expressed as a percentage of total Pax6+ nuclei. (c) Quantification of the percentage ofTis21-GFP+ (green) andTis21-GFP− (white) Tbr2−/Pax6+ nuclei in VZ+SVZ. (d,e) Pax6 (red), Tbr1 (d) or Tuj1 (e) (green) and DAPI (white) staining. Scale bar, 50 μm. (f) Tbr2 (red), Tbr1 (blue),Tis21-GFP (green) and DAPI (white) staining. Red arrowheads, Tbr2+/Tbr1−/Tis21-GFP+ nucleus (BP); yellow arrowheads, Tbr2+/Tbr1+/Tis21-GFP+ nucleus (neuron); blue arrowheads, Tbr2−/Tbr1+/Tis21-GFP+ nucleus (neuron). Scale bar, 50 μm. (g) Quantification of Tbr1+/Tbr2+ (blue–red) and Tbr1−/Tbr2+ (red) nuclei in VZ, SVZ and VZ+SVZ, each expressed as a percentage of total Tbr2+ nuclei. (h) Quantification of the percentage ofTis21-GFP+ (green) andTis21-GFP− (white) Tbr1−/Tbr2+ nuclei in VZ+SVZ. (a,d,e,f) White lines at margins, VZ and SVZ boundaries. (b,c,g,h) Data are the mean of three 225-μm-wide fields, each from a different brain and litter; error bars indicate s.e.m. Images in (a,d,f) and data in (b,c,g,h) are from embryos subjected to cumulative EdU labelling for 5 h (a,d), 1 h (f) and 5, 9 and 12 h (b,c,g,h; compareSupplementary Fig. S4). Figure 1: Classification of proliferative and neurogenic APs and BPs on the basis of differential marker expression. ( a ) Pax6 (red), Tbr2 (blue), Tis21 -GFP (green) and DAPI (white) staining. Red arrowheads, Pax6+/Tbr2−/ Tis21 -GFP− nuclei (APs); yellow arrowheads, Pax6+/Tbr2+/ Tis21 -GFP+ nuclei (BPs); blue arrowheads, Pax6−/Tbr2+/ Tis21 -GFP+ nucleus (BP). Scale bar, 50 μm. ( b ) Quantification of Tbr2+/Pax6+ (blue–red) and Tbr2−/Pax6+ (red) nuclei in VZ, SVZ and VZ+SVZ, each expressed as a percentage of total Pax6+ nuclei. ( c ) Quantification of the percentage of Tis21 -GFP+ (green) and Tis21 -GFP− (white) Tbr2−/Pax6+ nuclei in VZ+SVZ. ( d , e ) Pax6 (red), Tbr1 ( d ) or Tuj1 ( e ) (green) and DAPI (white) staining. Scale bar, 50 μm. ( f ) Tbr2 (red), Tbr1 (blue), Tis21 -GFP (green) and DAPI (white) staining. Red arrowheads, Tbr2+/Tbr1−/ Tis21 -GFP+ nucleus (BP); yellow arrowheads, Tbr2+/Tbr1+/ Tis21 -GFP+ nucleus (neuron); blue arrowheads, Tbr2−/Tbr1+/ Tis21 -GFP+ nucleus (neuron). Scale bar, 50 μm. ( g ) Quantification of Tbr1+/Tbr2+ (blue–red) and Tbr1−/Tbr2+ (red) nuclei in VZ, SVZ and VZ+SVZ, each expressed as a percentage of total Tbr2+ nuclei. ( h ) Quantification of the percentage of Tis21 -GFP+ (green) and Tis21 -GFP− (white) Tbr1−/Tbr2+ nuclei in VZ+SVZ. ( a , d , e , f ) White lines at margins, VZ and SVZ boundaries. ( b , c , g , h ) Data are the mean of three 225-μm-wide fields, each from a different brain and litter; error bars indicate s.e.m. Images in ( a , d , f ) and data in ( b , c , g , h ) are from embryos subjected to cumulative EdU labelling for 5 h ( a , d ), 1 h ( f ) and 5, 9 and 12 h ( b , c , g , h ; compare Supplementary Fig. S4 ). Full size image In the SVZ, 26% of interphase nuclei were Pax6+, although most of these nuclei exhibited a lower level of Pax6 immunoreactivity compared with VZ nuclei. The overwhelming majority (≈85%) of Pax6+ interphase nuclei in the SVZ were also Tbr2+ and hence belonged to newborn BPs, whereas ≈15% of the Pax6+ SVZ nuclei were Tbr2− ( Fig. 1b ) and presumably belonged to APs the interkinetic nuclear migration of which extended into the SVZ. Analysis of Tbr2−/Pax6+ nuclei in the VZ and SVZ for Tis21 -GFP expression showed that ≈40% of APs had switched to generating neurons or neurogenic BPs ( Fig. 1c ; Supplementary Fig. S2 ). In contrast to the partial overlap between the populations of Pax6+ and Tbr2+ nuclei, we observed very little (if any) overlap between the Pax6+ and Tbr1+ nuclei populations ( Fig. 1d ). This indicated that Pax6 expression, although extending into a portion of the BP population, did not significantly extend into the population of newborn neurons. Consistent with this conclusion, we observed very little (if any) immunostaining for βIII-tubulin (Tuj1), a marker of newborn neurons, in the VZ ( Fig. 1e ). With regard to BPs, in addition to the ≈30% fraction of interphase nuclei in the VZ, the vast majority (≈90%) of interphase nuclei in the SVZ were Tbr2+ ( Fig. 1f ). Counter immunofluorescence for Tbr1 revealed that <5% of the Tbr2+ interphase nuclei in the VZ were Tbr1+ ( Fig. 1g ), indicating that BPs contributed >95% to the Tbr2+ interphase nuclei in the VZ. In the SVZ, ≈40% of Tbr2+ nuclei were also Tbr1+ and hence belonged to newborn neurons, whereas ≈60% of the Tbr2+ interphase nuclei were Tbr1− ( Fig. 1g ) and hence BPs. Analysis of the Tbr1−/Tbr2+ nuclei in the VZ and SVZ for Tis21 -GFP expression showed that >80% of BPs were neurogenic ( Fig. 1h ). A summary of the population analysis in the VZ and SVZ is illustrated in Supplementary Figure S2 . BPs have a longer cell cycle than APs We next used the above information to determine the cell-cycle parameters of Tis21 -GFP-negative ( Tis21 -GFP−) and -positive ( Tis21 -GFP+) APs and BPs, using cumulative labelling with 5-ethynyl-2-deoxyuridine (EdU). As described in Supplementary Note S2 , it was appropriate to use EdU instead of 5-bromo-2-deoxyuridine (BrdU; Supplementary Figs S3 and S4 ). Cumulative EdU labelling was performed in conjunction with triple immunostaining for either Pax6, Tbr2 plus Tis21 -GFP ( Fig. 2a,b ) or Tbr2, Tbr1 plus Tis21 -GFP ( Fig. 2c,d ) to determine the cell-cycle parameters for APs (Tbr2−/Pax6+) and BPs (Tbr1−/Tbr2+), respectively, and to distinguish between proliferative ( Tis21 -GFP−) and neurogenic ( Tis21 -GFP+) NPC sub-populations. 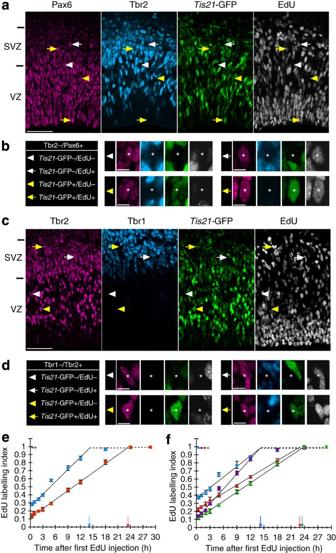Figure 2: Cumulative EdU labelling of proliferative and neurogenic APs and BPs. (a,b) Pax6 (magenta), Tbr2 (blue),Tis21-GFP (green) and EdU (white) staining after cumulative EdU labelling for 9 h. Individual AP nuclei indicated by arrows/arrowheads in (a) are shown at higher magnification in (b) (asterisks); white arrowheads, Pax6+/Tbr2−/Tis21-GFP−/EdU− nucleus; white arrows, Pax6+/Tbr2−/Tis21-GFP−/EdU+ nucleus; yellow arrowheads, Pax6+/Tbr2−/Tis21-GFP+/EdU− nucleus; yellow arrows, Pax6+/Tbr2−/Tis21-GFP+/EdU+ nucleus. VZ and SVZ are indicated on the left. Scale bars, 50 μm (a) and 10 μm (b). (c,d) Tbr2 (magenta), Tbr1 (blue),Tis21-GFP (green) and EdU (white) staining after cumulative EdU labelling for 9 h. Individual BP nuclei indicated by arrows/arrowheads in (c) are shown at higher magnification in (d) (asterisks); white arrowheads, Tbr2+/Tbr1−/Tis21-GFP−/EdU− nucleus; white arrows, Tbr2+/Tbr1−/Tis21-GFP−/EdU+ nucleus; yellow arrowheads, Tbr2+/Tbr1−/Tis21-GFP+/EdU− nucleus; yellow arrows, Tbr2+/Tbr1−/Tis21-GFP+/EdU+ nucleus. VZ and SVZ are indicated on the left. Scale bars, 50 μm (c) and 10 μm (d). (e,f) Proportion of EdU-labelled NPC nuclei (EdU labelling index) after cumulative EdU labelling for 0.5, 1, 2, 3, 5, 9, 12, 18, 24 and 29 h. The EdU labelling index was separately determined for the various AP (Pax6/Tbr2/GFP/EdU staining as in (a)) and BP (Tbr2/Tbr1/GFP/EdU staining as in (c)) populations, as follows: total APs (e, Tbr2−/Pax6+, blue circles), total BPs (e, Tbr1−/Tbr2+, red squares), proliferative APs (f, Tbr2−/Pax6+/Tis21-GFP−, blue diamonds), BP-genic/neurogenic APs (f, Tbr2−/Pax6+/Tis21-GFP+, purple squares), proliferative BPs (f, Tbr1−/Tbr2+/Tis21-GFP−, red triangles) and neurogenic BPs (f, Tbr1−/Tbr2+/Tis21-GFP+, green crosses). Data are the mean of three 225-μm-wide fields (except for the 1-, 9- and 29-h time points, which are from five, two and one field(s), respectively), each from a different brain and litter; error bars indicate s.e.m. or the range of the two individual values. Dashed lines and colour-coded arrowheads indicate the growth fraction; colour-coded arrows indicate the time point at which the labelling index reaches a plateau (TC–TS). As shown in Figure 2e and summarized in Table 1 , this revealed that the length of G2+M+G1 ( T C – T S ), as indicated by the time point at which the EdU labelling index reached the plateau, was longer for the total population of BPs (23.3 h) than APs (14.1 h). In contrast, the proportion of the cell cycle comprising S-phase, as indicated by the intercept of the cumulative EdU labelling curve with the y axis, was smaller for BPs (12%) than for APs (26%). The growth fraction was nearly 100% for both, APs and BPs. Calculation of the length of S-phase ( T S ) and the total cell cycle ( T C ) [24] yielded values of 5.0 and 19.1 h for APs and 3.2 and 26.5 h for BPs. The present T C data determined by cumulative EdU labelling are very similar to those determined by live imaging in organotypic slice culture [7] , [20] . Figure 2: Cumulative EdU labelling of proliferative and neurogenic APs and BPs. ( a , b ) Pax6 (magenta), Tbr2 (blue), Tis21 -GFP (green) and EdU (white) staining after cumulative EdU labelling for 9 h. Individual AP nuclei indicated by arrows/arrowheads in ( a ) are shown at higher magnification in ( b ) (asterisks); white arrowheads, Pax6+/Tbr2−/ Tis21 -GFP−/EdU− nucleus; white arrows, Pax6+/Tbr2−/ Tis21 -GFP−/EdU+ nucleus; yellow arrowheads, Pax6+/Tbr2−/ Tis21 -GFP+/EdU− nucleus; yellow arrows, Pax6+/Tbr2−/ Tis21 -GFP+/EdU+ nucleus. VZ and SVZ are indicated on the left. Scale bars, 50 μm ( a ) and 10 μm ( b ). ( c , d ) Tbr2 (magenta), Tbr1 (blue), Tis21 -GFP (green) and EdU (white) staining after cumulative EdU labelling for 9 h. Individual BP nuclei indicated by arrows/arrowheads in ( c ) are shown at higher magnification in ( d ) (asterisks); white arrowheads, Tbr2+/Tbr1−/ Tis21 -GFP−/EdU− nucleus; white arrows, Tbr2+/Tbr1−/ Tis21 -GFP−/EdU+ nucleus; yellow arrowheads, Tbr2+/Tbr1−/ Tis21 -GFP+/EdU− nucleus; yellow arrows, Tbr2+/Tbr1−/ Tis21 -GFP+/EdU+ nucleus. VZ and SVZ are indicated on the left. Scale bars, 50 μm ( c ) and 10 μm ( d ). ( e , f ) Proportion of EdU-labelled NPC nuclei (EdU labelling index) after cumulative EdU labelling for 0.5, 1, 2, 3, 5, 9, 12, 18, 24 and 29 h. The EdU labelling index was separately determined for the various AP (Pax6/Tbr2/GFP/EdU staining as in ( a )) and BP (Tbr2/Tbr1/GFP/EdU staining as in ( c )) populations, as follows: total APs ( e , Tbr2−/Pax6+, blue circles), total BPs ( e , Tbr1−/Tbr2+, red squares), proliferative APs ( f , Tbr2−/Pax6+/ Tis21 -GFP−, blue diamonds), BP-genic/neurogenic APs ( f , Tbr2−/Pax6+/ Tis21 -GFP+, purple squares), proliferative BPs ( f , Tbr1−/Tbr2+/ Tis21 -GFP−, red triangles) and neurogenic BPs ( f , Tbr1−/Tbr2+/ Tis21 -GFP+, green crosses). Data are the mean of three 225-μm-wide fields (except for the 1-, 9- and 29-h time points, which are from five, two and one field(s), respectively), each from a different brain and litter; error bars indicate s.e.m. or the range of the two individual values. Dashed lines and colour-coded arrowheads indicate the growth fraction; colour-coded arrows indicate the time point at which the labelling index reaches a plateau ( T C – T S ). Full size image Table 1 Cell-cycle parameters of Tis21 -GFP – and Tis21 -GFP + APs and BPs in E14.5 mouse neocortex. Full size table Proliferative NPCs have a longer S-phase than neurogenic NPCs We next analysed the cell-cycle parameters separately for Tis21 -GFP− APs and BPs, that is, those destined to undergo proliferative divisions [6] , and Tis21 -GFP+ APs and BPs, that is, those destined to undergo BP-genic (APs) and neurogenic (APs, BPs) divisions [6] , [9] ( Fig. 2f , Table 1 ). T C – T S was nearly identical for proliferative (14.1 h) and BP-genic/neurogenic (14.0 h) APs, and the same was the case for the longer T C – T S of proliferative (23.0 h) versus neurogenic (23.4 h) BPs. However, interestingly, the T S value of BP-genic/neurogenic APs and neurogenic BPs was significantly shorter (1.8 and 2.8 h, respectively) than that of proliferative APs and BPs (8.3 and 6.4 h, respectively). This resulted in a shorter T C of BP-genic/neurogenic APs (15.8 h) than of proliferative APs (22.4 h), and of neurogenic BPs (26.2 h) than of proliferative BPs (29.4 h). Given that the Tis21 -GFP+ sub-population is greater for BPs (>80%, Fig. 1h ) than for APs (≈40%, Fig. 1c ), the shorter S-phase duration of BP-genic/neurogenic compared with proliferative NPCs ( Fig. 2f ) contributed to the observation ( Fig. 2e ) that S-phase comprised a smaller proportion of the T C of BPs than of APs. We sought to corroborate the difference between APs and BPs with regard to the S-phase proportion relative to the total cell cycle by determining the proportion of NPCs in S-phase using an independent method, that is, proliferating cell nuclear antigen (PCNA) immunostaining. Cell nuclei in S-phase typically exhibit a punctate pattern of PCNA immunoreactivity, which reflects sites of DNA replication, whereas nuclei in G1 and G2 show diffuse PCNA immunoreactivity ( Fig. 3a–d ) [37] , [38] . Determination of the percentage of Pax6+ ( Fig. 3a ) and Tbr2+ ( Fig. 3b ) nuclei in S-phase by PCNA immunostaining, together with correction for the contribution of neurons to the Tbr2+ nuclei and of BPs to the Pax6+ nuclei ( Fig. 1b,g ) as described in the Methods, allowed us to calculate the percentage of APs and BPs in S-phase (30±4 and 14±4%, respectively; Fig. 3e ). 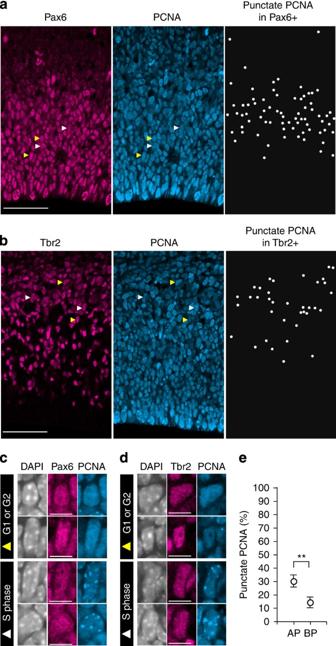Figure 3: Identification of S-phase NPC nuclei by PCNA immunostaining. (a,b,c,d) Pax6 (magenta) or Tbr2 (magenta), PCNA (blue) and DAPI staining (c,d, white). Individual nuclei indicated by arrowheads in (a) and (b) are shown at higher magnification in (c) and (d), respectively; white arrowheads, S-phase nuclei showing punctate PCNA immunoreactivity; yellow arrowheads, G1- or G2-phase nuclei showing homogeneous PCNA immunoreactivity. All Pax6+ nuclei (a) and all Tbr2+ nuclei (b) that show punctate PCNA immunoreactivity are indicated by white dots in the respective right panel. Scale bars, 50 μm (a,b) and 10 μm (c,d). (e) Percentage of AP and BP nuclei that are in S-phase as revealed by PCNA immunostaining. Data show the percentage value of (BP) total Tbr2+ nuclei in VZ+SVZ showing punctate PCNA immunoreactivity, corrected for the contribution of neurons, and of (AP) total Pax6+ nuclei in VZ+SVZ showing punctate PCNA immunoreactivity, corrected for the contribution of BPs, and are the mean of four 225-μm-wide fields, each from a different brain and litter; error bars indicate s.d.; **P<0.01. (a–e) Images in (a–d) and data in (e) are from embryos subjected to cumulative EdU labelling for 5 and 3–9 h, respectively. Very similar data to that shown in Figure 3e (EdU-labelled samples) were obtained when embryos not exposed to EdU were analysed (APs 26±6% ( n =3); BPs 12–14% ( n =2)). These data compare well with the mean proportion of NPCs in S-phase as determined from the intercept of the cumulative EdU-labelling curves with the y axis ( Fig. 2e ). Figure 3: Identification of S-phase NPC nuclei by PCNA immunostaining. ( a , b , c , d ) Pax6 (magenta) or Tbr2 (magenta), PCNA (blue) and DAPI staining ( c , d , white). Individual nuclei indicated by arrowheads in ( a ) and ( b ) are shown at higher magnification in ( c ) and ( d ), respectively; white arrowheads, S-phase nuclei showing punctate PCNA immunoreactivity; yellow arrowheads, G1- or G2-phase nuclei showing homogeneous PCNA immunoreactivity. All Pax6+ nuclei ( a ) and all Tbr2+ nuclei ( b ) that show punctate PCNA immunoreactivity are indicated by white dots in the respective right panel. Scale bars, 50 μm ( a , b ) and 10 μm ( c , d ). ( e ) Percentage of AP and BP nuclei that are in S-phase as revealed by PCNA immunostaining. Data show the percentage value of (BP) total Tbr2+ nuclei in VZ+SVZ showing punctate PCNA immunoreactivity, corrected for the contribution of neurons, and of (AP) total Pax6+ nuclei in VZ+SVZ showing punctate PCNA immunoreactivity, corrected for the contribution of BPs, and are the mean of four 225-μm-wide fields, each from a different brain and litter; error bars indicate s.d. ; ** P <0.01. ( a – e ) Images in ( a – d ) and data in ( e ) are from embryos subjected to cumulative EdU labelling for 5 and 3–9 h, respectively. Full size image Longer cell cycle of BPs than of APs is due to G1 lengthening We combined EdU labelling with immunostaining for phosphohistone H3 (PH3), an indicator of late G2- and M-phase [39] , to investigate the duration of G2 and M in the various NPC populations. PH3+ cells, the mitotic state (as opposed to late G2) of which was confirmed by 4,6-diamidino-2-phenylindole (DAPI) staining, were classified as either APs or BPs on the basis of their location at the ventricular surface or in the basal VZ/SVZ, respectively ( Fig. 4a,b ), and as undergoing proliferative or neurogenic division on the basis of the absence or presence, respectively, of Tis21 -GFP ( Fig. 4c,d ). 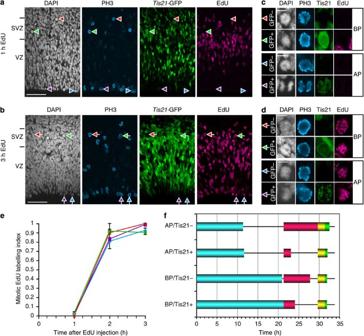Figure 4: Time course of appearance of EdU label in proliferative and neurogenic mitotic APs and BPs. (a–d) Phosphohistone H3 (PH3, blue),Tis21-GFP (green), DAPI (white) and EdU (magenta) staining after cumulative EdU labelling for 1 h (a,c) and 3 h (b,d). Examples of cells in mitosis, as identified by positive PH3 immunostaining (PH3+) plus mitotic appearance on DAPI staining (DAPI-m), are indicated by arrowheads in (a) and (b) and are shown at higher magnification in (c) and (d), respectively; red arrowheads, DAPI-m/PH3+/Tis21-GFP−/EdU− cell (BP); green arrowheads, DAPI-m/PH3+/Tis21-GFP+/EdU− cell (BP); blue arrowheads, DAPI-m/PH3+/Tis21-GFP−/EdU− cell (AP); purple arrowheads, DAPI-m/PH3+/Tis21-GFP+/EdU− cell (AP); red arrows, DAPI-m/PH3+/Tis21-GFP−/EdU+ cell (BP); green arrows, DAPI-m/PH3+/Tis21-GFP+/EdU+ cell (BP); blue arrows, DAPI-m/PH3+/Tis21-GFP−/EdU+ cell (AP); purple arrows, DAPI-m/PH3+/Tis21-GFP+/EdU+ cell (AP). VZ and SVZ are indicated on the left. Scale bars, 50 μm (a,b) and 10 μm (c,d). (e) Proportion of EdU-labelled mitotic cells (mitotic EdU labelling index) after cumulative EdU labelling for the indicated times. The mitotic EdU labelling index was separately determined for proliferative APs (apicalTis21-GFP− mitoses, blue diamonds), BP-genic/neurogenic APs (apicalTis21-GFP+ mitoses, purple squares), proliferative BPs (basalTis21-GFP− mitoses, red triangles) and neurogenic BPs (basalTis21-GFP+ mitoses, green crosses). Data are the mean of three (except 2 h: where the mean is of two fields) 450-μm wide fields (sum of two 225-μm fields), each from a different brain and litter; error bars indicate s.e.m. or the range of the two individual values. (f) Diagram showing the duration of the cell-cycle phases in each NPC population (seeTable 1). Blue bars, G1-phase; red bars, S-phase; yellow bars, G2-phase; green bars, M-phase. Figure 4: Time course of appearance of EdU label in proliferative and neurogenic mitotic APs and BPs. ( a – d ) Phosphohistone H3 (PH3, blue), Tis21 -GFP (green), DAPI (white) and EdU (magenta) staining after cumulative EdU labelling for 1 h ( a , c ) and 3 h ( b , d ). Examples of cells in mitosis, as identified by positive PH3 immunostaining (PH3+) plus mitotic appearance on DAPI staining (DAPI-m), are indicated by arrowheads in ( a ) and ( b ) and are shown at higher magnification in ( c ) and ( d ), respectively; red arrowheads, DAPI-m/PH3+/ Tis21 -GFP−/EdU− cell (BP); green arrowheads, DAPI-m/PH3+/ Tis21 -GFP+/EdU− cell (BP); blue arrowheads, DAPI-m/PH3+/ Tis21 -GFP−/EdU− cell (AP); purple arrowheads, DAPI-m/PH3+/ Tis21 -GFP+/EdU− cell (AP); red arrows, DAPI-m/PH3+/ Tis21 -GFP−/EdU+ cell (BP); green arrows, DAPI-m/PH3+/ Tis21 -GFP+/EdU+ cell (BP); blue arrows, DAPI-m/PH3+/ Tis21 -GFP−/EdU+ cell (AP); purple arrows, DAPI-m/PH3+/ Tis21 -GFP+/EdU+ cell (AP). VZ and SVZ are indicated on the left. Scale bars, 50 μm ( a , b ) and 10 μm ( c , d ). ( e ) Proportion of EdU-labelled mitotic cells (mitotic EdU labelling index) after cumulative EdU labelling for the indicated times. The mitotic EdU labelling index was separately determined for proliferative APs (apical Tis21 -GFP− mitoses, blue diamonds), BP-genic/neurogenic APs (apical Tis21 -GFP+ mitoses, purple squares), proliferative BPs (basal Tis21 -GFP− mitoses, red triangles) and neurogenic BPs (basal Tis21 -GFP+ mitoses, green crosses). Data are the mean of three (except 2 h: where the mean is of two fields) 450-μm wide fields (sum of two 225-μm fields), each from a different brain and litter; error bars indicate s.e.m. or the range of the two individual values. ( f ) Diagram showing the duration of the cell-cycle phases in each NPC population (see Table 1 ). Blue bars, G1-phase; red bars, S-phase; yellow bars, G2-phase; green bars, M-phase. Full size image Analysis of the appearance of EdU label in mitotic figures (mitotic EdU labelling index) revealed a very similar time course for the four NPC populations ( Fig. 4e ), with almost all mitotic NPCs becoming EdU+ 2–3 h after EdU administration, indicating an average G2-length ( T G2 ) of <2 h ( ∼ 1.6 h). With regard to M-phase, we first determined the percentages of total Tis21 -GFP− and Tis21 -GFP+ APs and BPs, identified as in Figure 1 , that were in M-phase by DAPI staining and PH3 immunofluorescence as in Figure 4a–d , and then calculated the length of M-phase ( T M ) in the four NPC populations from the respective T C . This revealed that T M was longer in APs than in BPs, being longest in Tis21 -GFP− APs ( Table 1 ). The determination of T C , T S , T G2 and T M allowed us to calculate the length of G1 ( T G1 ). T G1 was found to be almost twice as long for BPs than for APs, and for either type of NPC was not significantly different for the proliferative and BP-genic/neurogenic sub-populations (APs, 11.4 and 11.7 h, respectively; BPs, 20.9 and 21.3 h, respectively; Fig. 4f , Table 1 ). Higher DNA synthesis rate in Tis21 -GFP+ than in Tis21 -GFP− NPCs To investigate possible mechanisms underlying the S-phase shortening in Tis21 -GFP+ compared with Tis21 -GFP− NPCs, we performed EdU pulse-labelling for 30 min in vivo and analysed dissociated single Tis21 -GFP− and Tis21 -GFP+ NPCs, separated by fluorescence-activated cell sorting (FACS), by flow cytometry. Comparison of the overtly EdU-incorporating Tis21 -GFP− ( Fig. 5a , dashed line) and Tis21 -GFP+ ( Fig. 5b , dashed line) NPC populations revealed a 20% increase in the rate of EdU incorporation in Tis21 -GFP+ cells ( Fig. 5c ). This increase was corroborated when only the overtly EdU-incorporating NPCs in S-phase, as defined by DNA content ( Fig. 5d,e ), were quantified, and observed for cells in early and late S-phase ( Fig. 5f ; Fig. 5g,h for Tis21 -GFP−; Fig. 5i,j for Tis21 -GFP+). Thus, Tis21 -GFP+ NPCs exhibited a higher rate of DNA synthesis than Tis21 -GFP− NPCs, although the magnitude of this increase (1.2-fold change) was clearly less than that of the reduction in S-phase duration (3.3-fold change) in Tis21 -GFP+ compared with Tis21 -GFP− NPCs ( Fig. 4f , Table 1 , see Supplementary Fig. S2 for proportions of NPC sub-populations). 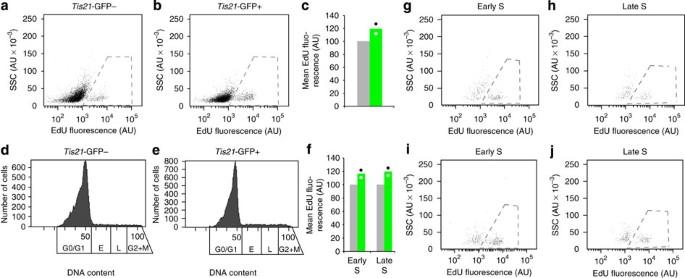Figure 5: Quantification of DNA synthesis rate by EdU incorporation inTis21-GFP− andTis21-GFP+ NPCs. Following a 30-min EdU pulse labelling (two litters), cortical cells were dissociated, analysed by flow cytometry and sorted forTis21-GFP fluorescence.Tis21-GFP− andTis21-GFP+ cells were then separately analysed for DNA content and EdU incorporation in another round of flow cytometry, as shown in the panels. (a,b) Granularity (side scatter, SSC; AU, arbitrary units) versus EdU fluorescence of singleTis21-GFP− (a, 8,053 cells) andTis21-GFP+ (b, 8,029 cells) cells. Dashed lines, overtly EdU-incorporating cells quantified in (c). Plots show one of the two litters analysed. (c) Mean EdU fluorescence of the overtly EdU-incorporating singleTis21-GFP− (grey column) andTis21-GFP+ (green column) cells. For each litter, the mean EdU fluorescence ofTis21-GFP− cells was arbitrarily set to 100, and the mean EdU fluorescence ofTis21-GFP+ cells was expressed relative to this. Data are the mean of two litters, dots indicate the two individual values. (d,e) Cell number versus DNA content of the singleTis21-GFP− (d) andTis21-GFP+ (e) cells shown in (a) and (b), respectively. Boxes indicate the sub-populations of cells in G0/G1, early S, late S and G2+M phases, as defined by DNA content; cells in early and late S-phases were analysed for SSC versus EdU fluorescence in (g–j). (f) Mean EdU fluorescence of the overtly EdU-incorporating singleTis21-GFP− (grey columns) andTis21-GFP+ (green columns) cells in early (g,i) and late (h,j) S-phase, as defined by DNA content (d,e) and after analysis of SSC versus EdU fluorescence (g–j). Quantification as in (c). (g–j) Granularity (SSC) versus EdU fluorescence of singleTis21-GFP− (g,h) andTis21-GFP+ (i,j) cells in early (g,i) and late (h,j) S phase shown in (d) and (e), respectively. Dashed lines, overtly EdU-incorporating cells quantified in (f). Plots show one of the two litters analysed. AU, arbitrary units. Figure 5: Quantification of DNA synthesis rate by EdU incorporation in Tis21 -GFP− and Tis21 -GFP+ NPCs. Following a 30-min EdU pulse labelling (two litters), cortical cells were dissociated, analysed by flow cytometry and sorted for Tis21 -GFP fluorescence. Tis21 -GFP− and Tis21 -GFP+ cells were then separately analysed for DNA content and EdU incorporation in another round of flow cytometry, as shown in the panels. ( a , b ) Granularity (side scatter, SSC; AU, arbitrary units) versus EdU fluorescence of single Tis21 -GFP− ( a , 8,053 cells) and Tis21 -GFP+ ( b , 8,029 cells) cells. Dashed lines, overtly EdU-incorporating cells quantified in ( c ). Plots show one of the two litters analysed. ( c ) Mean EdU fluorescence of the overtly EdU-incorporating single Tis21 -GFP− (grey column) and Tis21 -GFP+ (green column) cells. For each litter, the mean EdU fluorescence of Tis21 -GFP− cells was arbitrarily set to 100, and the mean EdU fluorescence of Tis21 -GFP+ cells was expressed relative to this. Data are the mean of two litters, dots indicate the two individual values. ( d , e ) Cell number versus DNA content of the single Tis21 -GFP− ( d ) and Tis21 -GFP+ ( e ) cells shown in ( a ) and ( b ), respectively. Boxes indicate the sub-populations of cells in G0/G1, early S, late S and G2+M phases, as defined by DNA content; cells in early and late S-phases were analysed for SSC versus EdU fluorescence in ( g – j ). ( f ) Mean EdU fluorescence of the overtly EdU-incorporating single Tis21 -GFP− (grey columns) and Tis21 -GFP+ (green columns) cells in early ( g , i ) and late ( h , j ) S-phase, as defined by DNA content ( d , e ) and after analysis of SSC versus EdU fluorescence ( g – j ). Quantification as in ( c ). ( g – j ) Granularity (SSC) versus EdU fluorescence of single Tis21 -GFP− ( g , h ) and Tis21 -GFP+ ( i , j ) cells in early ( g , i ) and late ( h , j ) S phase shown in ( d ) and ( e ), respectively. Dashed lines, overtly EdU-incorporating cells quantified in ( f ). Plots show one of the two litters analysed. AU, arbitrary units. Full size image Increased PCNA level in short S-phase duration nuclei We also analysed the intensity and sub-nuclear pattern of PCNA immunoreactivity in NPC populations with different S-phase durations. As high-resolution PCNA immunostaining was not compatible with detecting Tis21 -GFP (see Methods ), we combined it with Tbr2 immunofluorescence, reasoning that a Tbr2+ S-phase nucleus can be attributed to a BP and a Tbr2− S-phase nucleus to an AP. Given that S-phase in the total BP population is substantially shorter than in the total AP population (3.2 versus 5.0 h, Table 1 ), which reflects the fact that the BP population contains twice as many Tis21 -GFP+ NPCs as the AP population (80 versus 40%, Fig. 1c,h , Supplementary Fig. S2 ), comparison of PCNA immunostaining between Tbr2+ and Tbr2− nuclei may reveal differences in the DNA replication machinery that are related to alterations in S-phase duration. In accordance with previous observations with non-neural cells [40] , [41] , we considered the following: AP and BP nuclei exhibiting diffuse PCNA immunoreactivity to be in G1 or G2 (see Fig. 3c,d ); nuclei exhibiting numerous small PCNA puncta above the level of diffuse PCNA immunoreactivity to be in early S-phase ( Fig. 6a ); and nuclei exhibiting strong, occasionally clustered PCNA puncta well above the level of diffuse PCNA immunoreactivity to be in late S-phase ( Fig. 6b ). Quantification of the average PCNA immunofluorescence of a nucleus showed that this value extended over a certain range for both early ( Fig. 6c ) and late ( Fig. 6d ) S-phase nuclei. Plotting these values in ascending order for late S-phase nuclei revealed a significant difference between Tbr2− and Tbr2+ nuclei ( Fig. 6d ), with the mean value of Tbr2+ nuclei being 18% higher than that of Tbr2− nuclei ( Fig. 6e ), whereas no significant difference was observed between early S-phase Tbr2− and Tbr2+ nuclei ( Fig. 6c,e ). Thus, nuclei with, on average, a shorter S-phase (BPs) appear to maintain PCNA immunoreactivity at late S-phase at higher levels than nuclei with, on average, a longer S-phase (APs), although the magnitude of this increase (1.2-fold change) was less than that of the reduction in S-phase duration (1.6-fold change) in BPs relative to APs ( Table 1 , see Supplementary Fig. S2 for proportions of NPC sub-populations). Moreover, the s.d. of PCNA immunofluorescence between the pixels of a given nucleus was similar for Tbr2− and Tbr2+ nuclei in early S-phase, but was significantly higher for Tbr2+ than for Tbr2− nuclei in late S-phase ( Fig. 6f ). This suggested that the variability of clustered PCNA immunoreactivity at late S-phase was greater in nuclei with, on average, a shorter S-phase (BPs) than nuclei with, on average, a longer S-phase (APs). 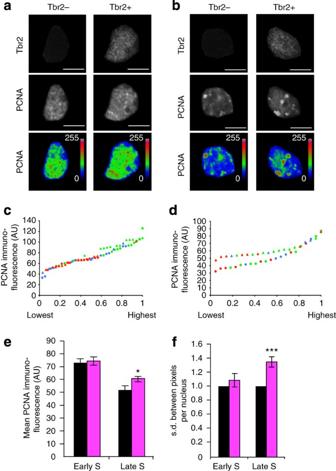Figure 6: Quantification of PCNA immunofluorescence in Tbr2− and Tbr2+ NPCs in early versus late S-phase. (a,b) Representative examples of PCNA immunofluorescence (white, middle panels, z-stack of five 0.95-μm optical sections from the centre of the nucleus) of Tbr2− (left panels) and Tbr2+ (right panels) NPCs. Nuclei showing relatively homogeneous PCNA immunoreactivity with a predominantly small punctate pattern were considered as early S-phase (a), nuclei showing a more heterogeneous PCNA immunoreactivity with a few strong clusters were considered as late S-phase (b). Intensity of PCNA immunofluorescence is shown in pseudocolour in the lower panels (blue, low values (0=lowest); red, high values (255=highest). Scale bars, 10 μm. (c–f) Quantification of PCNA immunofluorescence of Tbr2− and Tbr2+ NPCs in early and late S-phase as defined in (a) and (b), respectively. Data are from the same cryosection per embryo and are from three embryos, each from a different litter. Numbers of nuclei analysed for embryos 1, 2, 3, were Tbr2− early S (13, 14, 10), Tbr2+ early S (13, 12, 7), Tbr2− late S (8, 9, 5), Tbr2+ late S (8, 9, 4). (c,d) Average PCNA immunofluorescence (AU, arbitrary units) of individual Tbr2− (circles) and Tbr2+ (triangles) nuclei in early (c) and late (d) S-phase, plotted in order of increasing values, with the highest Tbr2− and Tbr2+ value arbitrarily set to 1. Red, green, blue symbols indicate embryos 1, 2, 3, respectively. Data distribution of Tbr2− versus Tbr2+ nuclei in late S-phase (d), Kolmogorov–SmirnovP-value=0.002. (e) Average PCNA immunofluorescence per nucleus of Tbr2− (black) and Tbr2+ (magenta) nuclei in early (left) and late (right) S-phase. Data are the mean of the values from the three embryos shown in (c) and (d); error bars, s.d.; *P=0.028. (f) s.d. of PCNA immunofluorescence between the pixels of a given nucleus. For each embryo, the mean s.d. of Tbr2− nuclei (black) in early (left) and late (right) S-phase was arbitrarily set to 1, and the mean s.d. of Tbr2+ nuclei (magenta) was expressed relative to this. Data are the mean of the three embryos; error bars, s.d.; ***P=0.001. Figure 6: Quantification of PCNA immunofluorescence in Tbr2− and Tbr2+ NPCs in early versus late S-phase. ( a , b ) Representative examples of PCNA immunofluorescence (white, middle panels, z-stack of five 0.95-μm optical sections from the centre of the nucleus) of Tbr2− (left panels) and Tbr2+ (right panels) NPCs. Nuclei showing relatively homogeneous PCNA immunoreactivity with a predominantly small punctate pattern were considered as early S-phase ( a ), nuclei showing a more heterogeneous PCNA immunoreactivity with a few strong clusters were considered as late S-phase ( b ). Intensity of PCNA immunofluorescence is shown in pseudocolour in the lower panels (blue, low values (0=lowest); red, high values (255=highest). Scale bars, 10 μm. ( c – f ) Quantification of PCNA immunofluorescence of Tbr2− and Tbr2+ NPCs in early and late S-phase as defined in ( a ) and ( b ), respectively. Data are from the same cryosection per embryo and are from three embryos, each from a different litter. Numbers of nuclei analysed for embryos 1, 2, 3, were Tbr2− early S (13, 14, 10), Tbr2+ early S (13, 12, 7), Tbr2− late S (8, 9, 5), Tbr2+ late S (8, 9, 4). ( c , d ) Average PCNA immunofluorescence (AU, arbitrary units) of individual Tbr2− (circles) and Tbr2+ (triangles) nuclei in early ( c ) and late ( d ) S-phase, plotted in order of increasing values, with the highest Tbr2− and Tbr2+ value arbitrarily set to 1. Red, green, blue symbols indicate embryos 1, 2, 3, respectively. Data distribution of Tbr2− versus Tbr2+ nuclei in late S-phase ( d ), Kolmogorov–Smirnov P -value=0.002. ( e ) Average PCNA immunofluorescence per nucleus of Tbr2− (black) and Tbr2+ (magenta) nuclei in early (left) and late (right) S-phase. Data are the mean of the values from the three embryos shown in ( c ) and ( d ); error bars, s.d. ; * P =0.028. ( f ) s.d. of PCNA immunofluorescence between the pixels of a given nucleus. For each embryo, the mean s.d. of Tbr2− nuclei (black) in early (left) and late (right) S-phase was arbitrarily set to 1, and the mean s.d. of Tbr2+ nuclei (magenta) was expressed relative to this. Data are the mean of the three embryos; error bars, s.d. ; *** P =0.001. Full size image Candidate genes for reducing S-phase duration of NPCs To gain further insight into the molecules possibly involved in these cell-cycle alterations, notably the S-phase shortening in Tis21 -GFP+ compared with Tis21 -GFP− NPCs, we carried out a genome-wide analysis of changes in mRNA levels. For this purpose, living Tis21 -GFP− and Tis21 -GFP+ NPCs in S-phase, as defined by DNA content, were isolated by FACS ( Supplementary Fig. S5 ) and subjected to microarray analysis. The FACS-based separation of Tis21 -GFP− and Tis21 -GFP+ NPCs was validated by analysis of mRNAs expected to be up- or down-regulated in these NPC populations ( Table 2 , see Supplementary Note S3 ). Table 2 mRNAs differentially expressed in FACS-isolated Tis21 -GFP+ versus Tis21 -GFP− S-phase NPCs of E14.5 mouse neocortex. Full size table Genome-wide analysis revealed 1,098 annotated mRNAs, the levels of which showed a statistically significant ( P <0.05) ≥1.2-fold change in Tis21 -GFP+ S-phase NPCs as compared with Tis21 -GFP−S-phase NPCs, with 410 mRNAs being upregulated and 688 mRNAs downregulated in Tis21 -GFP+ cells. Table 2 lists those among the 1,098 genes the functions of which suggested that they may be involved in the observed cell-cycle phase alterations, notably the 3.3-fold reduction in S-phase duration (from 8.0 to 2.4 h, Table 1 ), in Tis21 -GFP+ compared with Tis21 -GFP− NPCs. Indeed, alterations in mRNA levels were observed for genes involved in cell-cycle regulation and DNA replication and repair. Specifically, genes expected to be associated with a reduction in S-phase duration, such as the transcription factor E2f1 (refs 42 , 43 ), the phosphatase Cdc25a (ref. 44 ), cyclin G2 (ref. 45 ) and topoisomerase II alpha [46] , showed upregulated mRNA levels in Tis21 -GFP+ NPCs. Conversely, genes expected to be associated with an increase in S-phase duration, such as the repressor Erf [47] , [48] and the ubiquitin ligase complex subunit Fbxw7 (ref. 49 ), showed downregulated mRNA levels in Tis21 -GFP+ NPCs. We also observed an increase in the mRNA level of Cdk2ap1 (ref. 50 ), an inhibitor of G1/S transition, in Tis21 -GFP+ NPCs, consistent with the 1.3-fold increase in G1-phase duration (from 12.7 to 17.1 h, Table 1 ) in Tis21 -GFP+ compared with Tis21 -GFP− NPCs. However, mRNA levels of genes promoting G1/S transition, such as Cdk4 (ref. 51 ), were also upregulated. These functionally opposite changes in mRNA levels may reflect the fact that NPCs in S-phase had been isolated and subjected to microarray analysis. The reduction in S-phase duration in Tis21 -GFP+ compared with Tis21 -GFP− NPCs may also involve changes in gene expression that would affect the state of chromatin [52] , [53] . Indeed, we observed numerous such changes in mRNA levels, including genes involved in histone modification and DNA methylation. We also identified a number of genes implicated in NPC lineage progression, the mRNA levels of which were up- or down-regulated in Tis21 -GFP+ compared with Tis21 -GFP− NPCs ( Table 2 , Supplementary Note S4 ). Moreover, gene ontology (GO) term analysis ( Supplementary Table S1 , Supplementary Note S5 ) revealed that, remarkably, the downregulation of extracellular interactions is a major change that occurs in the transition from NPCs in S-phase destined to undergo proliferative divisions ( Tis21 -GFP−) to NPCs in S-phase destined to undergo differentiative divisions ( Tis21 -GFP+). Using cumulative EdU labelling and defining the various classes of NPCs using molecular markers rather than the location of their nuclei in histologically defined zones, our study provides the first detailed breakdown of cell-cycle parameters for the various classes of NPCs. The first key observation is that BPs have a substantially longer G1-phase than do APs. This may reflect, for example, that BPs delaminate from the apical adherens junction belt, translocate their nuclei over a greater distance in the basal direction (typically to the SVZ) than APs do in G1, and retract their apical and basal processes [5] , [7] , [9] . In addition, consistent with the cell-cycle length hypothesis [16] , [18] , this G1 lengthening may causally contribute to the more differentiated state of BPs compared with APs, and, perhaps, promote BP fate. Three implications of our data are addressed in the Supplementary Discussion : First, there is a need to reinterpret the previous observation [14] that Tis21 -GFP+ NPCs in the VZ have a longer G1 than do Tis21 -GFP− NPCs; second, the present finding of an equally long G2-phase in Tis21 -GFP+ APs and Tis21 -GFP+ BPs ( Fig. 4e , Table 1 ) is in contrast to a previous conclusion [14] that Tis21 -GFP+ BPs have a longer G2-phase than do Tis21 -GFP+ APs; third, the determination of T C of Tis21 -GFP+ BPs is valid. The second key observation is that self-expanding NPCs have on an average a 3.3-fold (range 2.3- to 4.6-fold) longer S-phase than NPCs committed to the neurogenic lineage. In fact, the key difference in cell-cycle parameters between proliferating and neurogenic NPCs is in S-phase duration, observed with two independent experimental approaches, whereas the other cell-cycle phases remain constant for proliferating versus neurogenic APs, and for proliferating versus neurogenic BPs. This finding raises the possibility that S-phase duration is a key factor in the maintenance of proliferative capacity of NPCs. Events in S-phase include DNA replication and repair coupled with cell-cycle checkpoints [54] , [55] . It has been reported that removal of Brca1 , a gene associated with DNA repair, causes massive apoptosis in early but not late NPCs [56] , suggesting a stronger requirement for the DNA repair system in proliferative compared with neurogenic NPCs. One may speculate that proliferative, more unrestricted NPCs (in terms of lineage) have a stronger requirement for DNA replication fidelity and repair, as errors would be inherited to many more progeny than errors in NPCs already restricted to differentiation [55] , [57] . Our data towards mechanistic insight into the change in S-phase duration are consistent with these considerations. First, determination of the rate of EdU incorporation revealed only an ≈20% increase in Tis21 -GFP+ compared with Tis21 -GFP− NPCs ( Fig. 5 ), indicating that DNA replication proceeded only a little more slowly in the latter cells and implying that their substantially longer S-phase was not due to a correspondingly lower rate of DNA synthesis. Second, in line with their 1.6-fold shorter S-phase ( Table 1 ), there was a 1.2-fold increase in PCNA immunoreactivity in BPs compared with APs, which was observed at late, but not early, S-phase, consistent with the activity of the DNA replication machinery remaining at a higher level in late S-phase in BPs compared with APs ( Fig. 6 ). Third, a genome-wide screen for changes in mRNA levels between Tis21 -GFP− and Tis21 -GFP+ NPCs in S-phase revealed several genes with key roles in cell-cycle regulation, DNA replication and repair and chromatin remodelling, the alterations in expression level of which provided possible mechanistic explanations for the difference in S-phase duration and its significance ( Table 2 ). Thus, we observed for S-phase Tis21 -GFP+ compared with Tis21 -GFP− NPCs an upregulation of genes implicated in increasing, and a downregulation of genes implicated in decreasing, S-phase duration; notably, the former included genes involved in the regulation of S-phase DNA checkpoints. Together, our data are consistent with the concept that the longer S-phase in Tis21 -GFP− compared with Tis21 -GFP+ NPCs reflects, for the most part, an increased time investment into the quality control of replicated DNA. It has previously been concluded [12] that S-phase duration in NPCs during cortical neurogenesis remains relatively constant. Our present finding that S-phase duration is dramatically different between proliferating and neurogenic NPCs has significant implications for studies in which conclusions about the extent of NPC proliferation are drawn from experiments using a single administration of thymidine analogues, notably BrdU. Thus, a lower proportion of BrdU-labelled cells observed after a single administration may not necessarily be indicative of a lower rate of cell proliferation, as commonly assumed, but may actually reflect a higher rate because of a reduction in S-phase duration. The present study delineates experimental approaches suitable to avoid such ambiguities. On a more general note, our study shows that cell-cycle regulation of NPCs, a key aspect of cortical development [16] , [17] , is more complex than previously assumed, involving major alterations not only in G1-phase but also in S-phase duration. The length of these cell-cycle phases seems to be differentially linked to NPC proliferation versus differentiation, with G1-phase lengthening being associated with the transition to a more differentiated NPC type, and maintenance of a long S-phase with NPC expansion. Animals Unless indicated otherwise, all mouse embryos used were E14.5 heterozygous Tis21 -GFP knock-in mice [6] (C57BL/6 background), obtained by overnight mating of homozygous Tis21 -GFP males with wild-type C57BL/6 females. Noon of the day on which the vaginal plug was observed was defined as embryonic day (E) 0.5. All animal studies were conducted in accordance with German animal welfare legislation and in strict pathogen-free conditions in the animal facility of the Max Planck Institute of Molecular Cell Biology and Genetics, Dresden, Germany. Protocols were approved by the Institutional Animal Welfare Officer (Tierschutzbeauftragter), and necessary licenses were obtained from the regional Ethical Commission for Animal Experimentation of Dresden, Germany (Tierversuchskommission, Landesdirektion Dresden). EdU labelling Cumulative EdU labelling was carried out by intraperitoneal injections, repeated at 3-h intervals up to 27 h, of 100 μl of 1 mg ml −1 EdU (Invitrogen) in PBS into pregnant mice (27–32 g) carrying E14.5 embryos, corresponding to ≈3.3 mg kg −1 of pregnant mouse. Mice were killed at the time points indicated in figures and legends, and the embryo-containing uteri were transferred to ice-cold PBS to stop further incorporation of EdU. In the case of comparison of cumulative BrdU and cumulative EdU labelling, 100–120 μl of 10 mg ml −1 BrdU (Sigma) in PBS, corresponding to 33–40 mg kg −1 of pregnant mouse, was coinjected with EdU, administered as above. For FACS analysis, pregnant mice carrying E14.5 embryos were killed 30 min after a single EdU injection as above, and the embryo-containing uteri were transferred to ice-cold Tyrode's solution to stop further incorporation of EdU. Immunofluorescence and EdU staining Immunofluorescence and EdU staining were performed on 10-μm transverse cryosections of dorsal telencephalon prepared from paraformaldehyde-fixed heads of E14.5 embryos, subjected to cumulative EdU labelling as indicated. For details, see Supplementary Methods . Unless indicated otherwise, images are 1.2-μm optical sections. Analysis of cell-cycle parameters For each of the NPC populations analysed (total APs, Tbr2−/Pax6+; total BPs, Tbr1−/Tbr2+; proliferative APs, Tbr2−/Pax6+/ Tis21 -GFP−; neurogenic APs, Tbr2−/Pax6+/ Tis21 -GFP+; proliferative BPs, Tbr1−/Tbr2+/ Tis21 -GFP−; neurogenic BPs, Tbr1−/Tbr2+/ Tis21 -GFP+), the proportional values of EdU-positive nuclei obtained after the various times of cumulative labelling (EdU labelling index) were used to determine the following cell-cycle parameters, using the Excel sheet provided by Dr R. Nowakowski [24] : the growth fraction, the proportion of total cell cycle covered by S-phase, T C – T S , T C and T S . The EdU labelling index curves were plotted using the Nowakowski Excel sheet. For estimating T G2 , we first defined NPCs as being in a mitotic state if this was revealed by both PH3 immunofluorescence and DAPI staining. Mitotic figures within three nuclear diameters from the ventricular surface were considered mitotic APs; mitotic figures in the basal half of the VZ and in the SVZ were considered mitotic BPs. The time required for half-maximal appearance of EdU label in the various mitotic AP and BP populations was taken to indicate the average T G2 . T M was calculated after determining the proportion of APs and BPs that were in mitosis, as identified by PH3 immunofluorescence and/or DAPI staining, taking into account the total cell-cycle length as determined by cumulative EdU labelling. Numbers of mitotic NPCs/total NPCs were as follows: total APs 372/7,832, Tis21 -GFP− APs 234/4,677, Tis21 -GFP+ APs 138/3,155, total BPs 130/6,803, Tis21 -GFP− BPs 19/1,037, Tis21 -GFP+ BPs 111/5,766; data are from 16 (mitotic APs and BPs), 17 (total APs) and 18 (total BPs) 225-μm-wide fields. The T C , T S , T G2 and T M values were then used to calculate T G1 of the respective NPC population. Determination of the percentage of S-phase nuclei by PCNA immunostaining The antigen retrieval protocol necessary to obtain high-resolution PCNA immunostaining such as that shown in Figure 3c,d was not compatible with detecting Tis21 -GFP by immunofluorescence, and did not yield high-quality PCNA images when combined with the present transcription factor double immunofluorescence protocol as used in Figure 1a,f , but allowed only single transcription factor immunofluorescence. We therefore used the following approach to quantify the proportion of APs and BPs in S-phase using the pattern of PCNA immunostaining. We first determined the percentage of total Pax6+ ( Fig. 3a ) and total Tbr2+ ( Fig. 3b ) nuclei that were in S-phase. The percentage value for the Tbr2+ S-phase nuclei obtained (11±3%, n =4, Fig. 3b ) was then corrected for the contribution of neurons (22±1%, see Fig. 1g , VZ+SVZ, blue–red portion of the column), assumed to have no S-phase, to yield the percentage of BPs in S-phase (14±4%, n =4, Fig. 3e ). Next, the latter value was used to correct the percentage value obtained for Pax6+ S-phase nuclei (23±2%, n =4, Fig. 3a ) for the contribution of BPs (37±2%, see Fig. 1b , VZ+SVZ, blue–red portion of column) in S-phase, to obtain the percentage of APs in S-phase (30±4%, n =4, Fig. 3e ). Quantification of PCNA immunofluorescence of S-phase cells PCNA immunofluorescence in Tbr2− and Tbr2+ S-phase nuclei was quantified using the previously described ImageJ macro [58] , which allows for an unbiased, fluorescence intensity-based definition of nuclear area. For each nucleus, the average PCNA immunofluorescence was the sum of the values of each pixel divided by the number of pixels of that nucleus, with subtraction of a background value (determined in the extracellular area). The macro also yielded the s.d. of the PCNA immunofluorescence signal between the pixels of a given nucleus. Flow cytometry and FACS Dorsal telencephalon (cerebral cortex) was dissected from E14.5 Tis21 -GFP knock-in embryos in ice-cold Tyrode's solution. Dissected tissue from three embryos (one litter) was minced using a pair of small forceps and incubated for 20 min at 37 °C in 700 μl of a 1:1 mixture of DMEM and Ham's F-12 (Invitrogen) containing 0.13% (w/v) DPCC-treated trypsin (Sigma, T1005), 0.067% (w/v) hyaluronidase (Sigma, H3884) and 0.02% (w/v) kynurenic acid (Sigma, K3375), followed by addition of 0.07% (w/v) soybean trypsin inhibitor (Sigma, T6522) in 700 μl of DMEM/Ham's F-12. Tissue pieces and cells were collected by centrifugation at 600 g for 5 min and resuspended in 700 μl of DMEM/Ham's F-12 containing 0.07% (w/v) trypsin inhibitor. The cells were dissociated by gentle trituration (10–20 up-and-down passages using a P-1000 tip), collected by centrifugation at 600 g for 5 min and resuspended in 500 μl of DMEM/Ham's F-12. The cell suspension was then passed through a filter (20-μm pore size, BD Bioscience) including a 500-μl rinse with DMEM/Ham's F-12 to obtain ≈1 ml of a suspension enriched in single cells (≈6×10 5 ). For the determination of EdU incorporation into Tis21 -GFP− and Tis21 -GFP+ NPCs, an aliquot of the cell suspension containing ≈10 4 cells was first analysed by flow cytometry using a FACSAria II cell sorter (BD Bioscience, run in PBS) and FACSDiva software to determine the range of Tis21 -GFP fluorescence. For comparison, cells from E14.5 wild-type embryos not subjected to EdU labelling were analysed (see Supplementary Fig. S5a ). Cells with a fluorescence value >1.05×10 3 U were defined as Tis21 -GFP+ and cells with a fluorescence value <8×10 2 U (AU, arbitrary units) were defined as Tis21 -GFP− (see Supplementary Fig. S5b ). Single cells (as defined by particle size, see Supplementary Fig. S5c ) were then sorted at room temperature to obtain ≈2×10 5 Tis21 -GFP− and Tis21 -GFP+ cells each. Subsequent flow cytometry of an aliquot of the sorted cell suspensions revealed that Tis21 -GFP− cells did not contain detectable numbers of cells with a fluorescence value >1×10 3 U, and the contribution of cells with a fluorescence value >1×10 3 U (AU) to the Tis21 -GFP+ cells was 99.5±2%. Sorted Tis21 -GFP− and Tis21 -GFP+ cells were separately processed using the Click-iT EdU Flow Cytometry Assay Kit with Alexa Fluor 647 for EdU detection, in combination with Click-iT EdU CellCycle 405-blue for DNA content determination (Invitrogen), according to the manufacturer's instructions, followed by another round of flow cytometry of the fixed and stained cells to define the populations of overtly EdU-incorporating cells and of cells in early or late S-phase, and to measure the amount of EdU incorporation into these cells. For microarray analysis, filtered cells obtained from the dorsal telencephalon of E14.5 Tis21 -GFP knock-in embryos as above were incubated for 1 h at 37 °C with a vital DNA dye (2 μl of Vybrant DyeCycle Violet Stain, Invitrogen). Live cells were analysed by flow cytometry to identify the population in S-phase on the basis of the level of DNA fluorescence (see Supplementary Fig. S5d,e ), and single live cells were then sorted to collect Tis21 -GFP− and Tis21 -GFP+ NPCs in S-phase cells, using the above FACS settings, which yielded 1–4×10 4 cells each per FACS run. The sorted cell suspensions were centrifuged at 600 g for 5 min, the supernatant discarded and cell pellets frozen in liquid nitrogen and stored at −80 °C. Microarray analysis Cell pellets of Tis21 -GFP− and Tis21 -GFP+ NPCs in S-phase were thawed in 102 μl of lysis buffer supplied with a total RNA isolation kit (NucleoSpin RNA XS, Macherey-Nagel). The cell lysate from one cell pellet was used consecutively to thaw the next cell pellet until a cell lysate corresponding to 1.5–2.0×10 5 cells was obtained. Total RNA was extracted using the NucleoSpin RNA XS kit according to the manufacturer's instructions. RNA from three independent experiments was used to perform One-Color Microarray-Based Gene Expression Analysis according to the manufacturer's instructions (Agilent Technologies). For each sample, 50 ng total RNA was used to prepare Cy3-labelled target cRNA with the Low Input Quick Amp Labeling Kit (Agilent Technologies). The target cRNAs were hybridized to SurePrint G3 Mouse GE 8×60K Microarrays (AMADID 028005, Agilent Technologies). Scanned images were analysed with Feature Extraction software 10.7.1.1 (Agilent Technologies) using default parameters (protocol: GE1_107_Sep09, grid: 028005_D_F_20100617) to obtain background-corrected signal intensities. The data were further analysed with GeneSpring GX Software (Version 11.0, Agilent Technologies). After quantile normalization of the data and removal of unreliable signal intensities (filtering of data by expression: in three out of six experiments the signal intensity of a probe had to be above the 20th percentile to be retained in the data set), mRNAs were considered differentially expressed in Tis21 -GFP+ versus Tis21 -GFP− cells if they had a corrected P -value <0.05 after an unpaired t -test and multiple testing correction (Benjamini Hochberg). GO term analysis of the differentially expressed mRNAs was performed with GeneSpring GX software, using a corrected P -value cutoff of <0.05 to define a GO term as being significantly increased or decreased in frequency as compared with the total population of mRNAs represented on the microarray. Statistical analyses P -values were determined using Student's t -test (two-sample equal variance, two tails). When indicated, the Kolmogorov–Smirnov test was used instead. Data deposition: The microarray data have been deposited in the NCBI Gene Expression Omnibus ( http://www.ncbi.nlm.nih.gov/geo/ ) with accession number GSE23585 . How to cite this article: Arai, Y. et al . Neural stem and progenitor cells shorten S-phase on commitment to neuron production. Nat. Commun. 2:154 doi: 10.1038/ncomms1155 (2011).